Surface modification-induced phase transformation of hexagonal close-packed gold square sheets Conventionally, the phase transformation of inorganic nanocrystals is realized under extreme conditions (for example, high temperature or high pressure). Here we report the complete phase transformation of Au square sheets (AuSSs) from hexagonal close-packed (hcp) to face-centered cubic (fcc) structures at ambient conditions via surface ligand exchange, resulting in the formation of (100) f -oriented fcc AuSSs. Importantly, the phase transformation can also be realized through the coating of a thin metal film (for example, Ag) on hcp AuSSs. Depending on the surfactants used during the metal coating process, two transformation pathways are observed, leading to the formation of (100) f -oriented fcc Au@Ag core-shell square sheets and (110) h /(101) f -oriented hcp/fcc mixed Au@Ag nanosheets. Furthermore, monochromated electron energy loss spectroscopy reveals the strong surface plasmon resonance absorption of fcc AuSS and Au@Ag square sheet in the infrared region. Our findings may offer a new route for the crystal-phase and shape-controlled synthesis of inorganic nanocrystals. In the past two decades, inorganic nanocrystals have been extensively studied because of their potential applications in catalysis [1] , energy conversion [2] , surface enhanced Raman scattering [3] and so on. The functional properties of inorganic nanocrystals can be tuned by controlling their size, shape, composition and topology [3] , [4] . In addition, the crystal phase of inorganic nanomaterials can also strongly affect their properties, such as magnetic [5] , [6] , optical [7] , catalytic [8] and electrical properties [9] . For instance, the phase transformation of FePt nanoparticles from face-centered cubic (fcc) to face-centered tetragonal structures led to the improved catalytic activity and durability for the oxygen reduction reaction [8] . Therefore, the study of crystal polymorphs and phase transformations of inorganic nanocrystals is essential to their controlled synthesis and wide applications. Conventionally, the phase transformation of inorganic nanocrystals is realized under high pressure [7] , [10] , [11] , [12] or at an elevated temperature [6] , [8] , [13] . In addition, the electron beam-induced phase transformation has also been observed, such as the transformation of Cu 2 S nanorods from low-chalcocite to high-chalcocite structures [14] . Meanwhile, cation exchange has also been used for the structure manipulation of inorganic nanocrystals [15] , [16] , [17] . However, it should be noted that the composition of the initial nanocrystals will be changed after the cation exchange. For instance, hexagonal CdSe nanocrytals can be transformed to cubic Ag 2 Se nanocrystals after cation exchange of Cd 2+ with Ag + ions [15] . Importantly, below a critical size, when the surface energy of a nanostructure dominates the total systemic energy, surfactant or solvent molecules can play a critical role in modulating its crystal structure [18] , [19] . For example, the surface of 3-nm ZnS nanoparticles synthesized in methanol underwent a transition from the disordered to the ordered cubic structure on bonding with water on surface [19] . However, until now it remains a great challenge to realize the complete transformation of a nanocrystal from one crystal phase to another at ambient conditions. The phase transformation of metals and alloys with close-packed structures (that is, hexagonal close-packed (hcp) or fcc) has been well studied both experimentally and theoretically [20] , [21] , [22] . The hcp and fcc polytypes differ from the stacking sequence of the close-packed planes with repeated ABABAB stacking along the [001] h direction and ABCABC stacking along the [111] f direction, respectively. In most cases, the hcp-to-fcc transformation in metals (for example, structural change of Co happens on annealing) is realized by the motion of partial dislocations on closed-packed planes, leading to the formation of stacking faults/twins or the mixed packing of hcp and fcc lattice planes [20] , [21] . To date, other phase transformation pathways/mechanisms between hcp and fcc structures have rarely been observed in noble metals [23] . In addition, surface plasmon resonance (SPR) property of metal nanostructures, especially nanoplates and nanosheets, has attracted great research interest due to their strong SPR absorption in the visible-infrared region, which can soundly benefit their various important applications (for example, infrared photothermal therapy) [1] , [3] , [24] , [25] . Conventionally, the SPR property of metal nanostructures is investigated by optical spectrophotometer. However, the spatial resolution of optical spectrophotometer is very low, and thus not suitable for the nanometre-scale plasmon characterization of individual metal nanostructures. Fortunately, with the recent development of monochromated electron energy loss spectroscopy (EELS) technique [26] , [27] , which combines high spatial and spectral resolution, the SPR property of an individual metal nanostructure can be measured. Recently, our group synthesized ultrathin Au square sheets (AuSSs) with the pure hcp structure, which are stable at ambient conditions [28] . Herein, we report that the AuSSs can be transformed from hcp to fcc structures via surface ligand exchange or surface coating of a thin metal layer (for example, Ag) at ambient conditions. The ligand exchange of hcp AuSSs leads to the formation of ultrathin fcc AuSSs with (100) f orientation. The surface coating, on the other hand, can lead to two types of phase transformation based on the different surfactants used, resulting in the formation of fcc Au@Ag core-shell square sheets with (100) f orientation, and hcp/fcc mixed Au@Ag core-shell nanosheets with (110) h /(101) f orientation. Moreover, the SPR properties of a single fcc AuSS or Au@Ag square sheet on graphene oxide (GO) are also studied by monochromated EELS. Synthesis of hcp AuSSs The hcp AuSSs capped by oleylamine were synthesized by our recently reported method with a slight modification [28] . In brief, hcp AuSSs were obtained by heating a growth solution consisting of HAuCl 4 (7.25 mM), oleylamine (150 mM), GO, hexane and ethanol at 58 °C for 16 h (see details in the Methods). The obtained AuSSs have an edge length of 100–500 nm, and thickness of 2.3±0.5 nm ( Supplementary Figs 1 and 2 ). Transmission electron microscope (TEM) analysis confirmed that the AuSSs have a pure hcp structure, consistent with our previous report ( Supplementary Fig. 1 ) [28] . Note that despite the fact that the fcc structure is more stable than the hcp one in the bulk gold, the ultrathin hcp AuSS is very stable in solution for at least several months at ambient conditions, because its low surface energy, due to the interaction with capping agent (oleylamine), dominates its total systemic energy [29] and thus stabilizes the hcp structure. Ligand exchange-induced phase transformation of hcp AuSSs The oleylamine initially capped on AuSSs can be exchanged by octadecanethiol (ODT) after the purified AuSS solution was mixed with a fresh ODT solution in hexane, which was then vortexed for 5 min at ambient conditions (see the Supplementary Information for details). The energy-dispersive X-ray spectroscopy (EDS) analysis ( Supplementary Fig. 3 ) and the X-ray photoelectron spectroscopy (XPS) data ( Supplementary Fig. 4 ) of the resulting product after purification confirmed that the oleylamine was exchanged by ODT, which was in agreement with the previous report [30] . The detailed TEM characterization of AuSSs after the ligand exchange, that is, oleylamine was exchanged by ODT, is shown in Fig. 1 . The square shape of AuSSs is preserved after the ligand exchange ( Fig. 1a,b ). Surprisingly, the crystal structure of the AuSS was completely transformed from hcp to fcc after the ligand exchange as verified by the selected area electron diffraction (SAED) patterns taken along two different zone axes ( Fig. 1c,d ). The SAED pattern of an AuSS lying flatly on a copper grid revealed a [100] f zone pattern ( Fig. 1c ), along with the other two diffraction rings attributed to {100} and {110} planes of GO, respectively. The SAED pattern along the [310] f zone axis ( Fig. 1d ) was also collected by tilting the fcc AuSSs around the [001] f zone axis for about 18.3°, which matches well with the theoretical angle (18.4°) between [100] f and [310] f zone axes, further confirming the fcc structure of as-obtained AuSSs. It is worth noting that the forbidden {011} f spots were observed in the SAED patterns of the fcc AuSS ( Fig. 1c,d ), suggesting a possible c(2 × 2) surface structure of thiol molecules adsorbed on the Au(100) f surface, which is consistent with the previous report [31] . High-resolution TEM (HRTEM) images of the fcc AuSS ( Fig. 1e,f ) show a square lattice pattern with an inter-plane spacing of 2.0 Å, assignable to {002} f planes. In addition, the high angular annular dark-field (HAADF)–scanning TEM (STEM) image of the cross-section of an fcc AuSS ( Fig. 1g ), which was cut by focused ion beam (FIB) along one of its diagonals, reveals a thickness of 3.1±0.5 nm ( Fig. 1h,i ). This is ~1.7 nm thinner than the thickness measured by atomic force microscopy (~4.8 nm, Supplementary Fig. 5 ), due to the surface adsorbed ODT molecules. The resulting fcc AuSS (3.1±0.5 nm in thickness) is ~35% thicker than the initial hcp AuSS (2.3±0.5 nm in thickness), which is consistent with the enlarged spacing between the atomic layers parallel to the basal plane, that is, from the initial d (110)h =1.5 Å to the final d (200)f =2.0 Å. High-resolution HAADF–STEM images taken in the centre ( Fig. 1h ) and on the edge ( Fig. 1i ) areas of the cross-section of the fcc AuSS show the [010] f zone lattice pattern, further confirming the complete phase transformation of AuSS from the hcp to fcc structure. 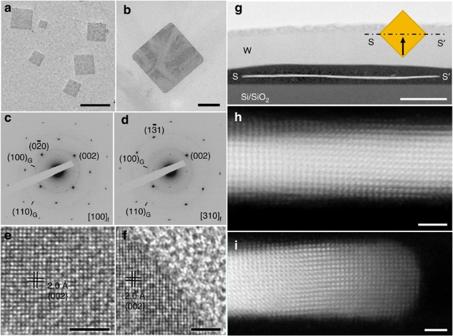Figure 1: TEM characterization of the obtained fcc AuSSs. (a) Low-magnification TEM image of fcc AuSSs (scale bar, 400 nm). (b) High-magnification TEM image of a typical fcc AuSS (Scale bar, 100 nm). (c) SAED pattern of a typical fcc AuSS taken along the [100]fzone axis. (d) SAED pattern of the [310]fzone axis acquired by tilting an fcc AuSS around the [001]fzone axis by 18.3° with respect to the [100]fzone axis. (e,f) HRTEM images of the centre and edge regions of fcc AuSSs, respectively (scale bars, 2 nm). (g) Low-magnification HAADF–STEM image showing the cross-section of an fcc AuSS that was prepared by FIB (scale bar, 100 nm). A tungsten (W) layer was deposited on top of the AuSS lying on a Si/SiO2substrate. Inset: schematic illustration showing that the cross-section was prepared by cutting the fcc AuSS along one of its diagonals; the arrow indicating the view direction of the cross-sectional STEM images. (h,i) High-resolution HAADF–STEM images (scale bars, 1 nm) showing the centre and edge regions of the cross-section of fcc AuSS ing. Figure 1: TEM characterization of the obtained fcc AuSSs. ( a ) Low-magnification TEM image of fcc AuSSs (scale bar, 400 nm). ( b ) High-magnification TEM image of a typical fcc AuSS (Scale bar, 100 nm). ( c ) SAED pattern of a typical fcc AuSS taken along the [100] f zone axis. ( d ) SAED pattern of the [310] f zone axis acquired by tilting an fcc AuSS around the [001] f zone axis by 18.3° with respect to the [100] f zone axis. ( e , f ) HRTEM images of the centre and edge regions of fcc AuSSs, respectively (scale bars, 2 nm). ( g ) Low-magnification HAADF–STEM image showing the cross-section of an fcc AuSS that was prepared by FIB (scale bar, 100 nm). A tungsten (W) layer was deposited on top of the AuSS lying on a Si/SiO 2 substrate. Inset: schematic illustration showing that the cross-section was prepared by cutting the fcc AuSS along one of its diagonals; the arrow indicating the view direction of the cross-sectional STEM images. ( h , i ) High-resolution HAADF–STEM images (scale bars, 1 nm) showing the centre and edge regions of the cross-section of fcc AuSS in g . Full size image Meanwhile, it was observed that the phase transformation of AuSSs is quite sensitive to the concentration of ODT ( Supplementary Figs 6 and 7 ). At relatively low ODT concentrations (for example, C ODT <20 mM), the ligand exchange led to the formation of irregularly shaped Au nanostructures with poor crystallinity ( Supplementary Fig. 6 ), whereas at higher ODT concentrations (typically, C ODT ≥20 mM) Au nanosheets with well-preserved square morphology and good crystallinity were obtained ( Supplementary Fig. 7 ). Note that in the aforementioned experiments, the concentration of Au atoms was kept constant (~2.3 mM). If the concentration of Au atoms was increased substantially (for example, 92 mM), while the ODT concentration was kept constant (25 mM), the complete phase transformation of AuSSs was also achieved ( Supplementary Fig. 8 ). These observations indicate that the sufficiently high concentration of ODT molecules in the solution ensured a rapid and complete exchange of oleylamine with ODT, and thus a uniform phase transformation over the entire structure of hcp AuSS. Besides ODT, other thiol molecules have also been used for the ligand exchange (the chemical structures of used thiols are shown in Supplementary Fig. 9 ). Our results ( Supplementary Fig. 10 ) demonstrated that the phase transformation of AuSSs can be achieved by various kinds of thiols, regardless of the length of n -alkane chain (3≤ n ≤18), hydrophilicity, the functional groups (for example, benzene, carboxylic acid or hydroxide), and the number of thiol groups (for example, monothiol or dithiol). The effects of thiols and other sulfur-containing species (for example, sulfur (S) and H 2 S) on the surface structure of metals have been studied previously [30] , [32] , [33] , [34] . It has been well documented that thiol molecules can induce surface reconstruction of gold films, for example, Au(111), due to the spontaneous formation of Au-S covalent bond [30] , [35] , [36] , [37] . In addition, other surface adsorbates like S have also been reported to cause surface reconstruction of metal films, particularly, favouring the formation of overlayers with high coordination numbers, such as fcc(100) that has a fourfold hollow site [34] . For example, S can induce the formation of a pseudo Ni{100} f –c(2 × 2)S overlayer structure, in which S atoms occupy the rectangular hollow sites of the pseudo Ni{100} f layer, on a Ni(111) f substrate [33] , [38] . Moreover, H 2 S can cause the faceting of spherical Pt nanoparticles to {100} f enclosed structures [39] . Therefore, the ligand exchange-induced phase transition of AuSS is likely initiated by a (100) f surface reconstruction induced by the adsorbed thiol molecules, followed by a complete phase transition over its entire structure. Metal coating-induced phase transformation of hcp AuSSs Importantly, besides the ligand exchange-induced phase transformation of AuSSs from pure hcp to fcc structures, we found that the phase transition of hcp AuSSs can also be achieved via coating a thin layer of metal film onto their surface. For example, we first coated Ag on hcp AuSSs by reducing AgNO 3 with L -ascorbic acid or NaBH 4 ( Fig. 2 and Supplementary Fig. 11 ). It can be seen that after coating of Ag, the square shape of the structures remained unchanged ( Fig. 2a ). The composition of the obtained Au–Ag square sheets was confirmed by EDS analysis ( Fig. 2f–h ; Supplementary Figs 12 and 13 ), which indicate the homogeneous distribution of Au and Ag in the bimetallic structures. Meanwhile, the XPS data reveal the obtained Au–Ag nanosheets are capped by oleylamine molecules ( Supplementary Fig. 14 ). The cross-sections of the Au–Ag bimetallic nanosheets were also prepared by FIB and analysed under TEM. Both EDS mapping ( Fig. 2i ) and line scanning ( Supplementary Fig. 15 ) of the cross-section of the bimetallic nanosheets suggested that the resulting products are Au@Ag core-shell structures. Depending on the amount of Ag deposited on hcp AuSSs, the thickness of the Au@Ag nanosheets varied from 3.0 to 4.6 nm ( Fig. 2i , Supplementary Figs 15–17 ). To our great surprise, SAED patterns ( Fig. 2b,c ) and HRTEM images ( Fig. 2d,e ) of such a nanosheet lying on a copper grid and the HAADF–STEM image of the cross-section of a nanosheet ( Fig. 2i ) indicate that the crystal structure of the Au@Ag square sheets is pure fcc with the (100) f orientation, similar to the structure of fcc AuSS obtained after ligand exchange ( Fig. 1 ). Note that the lattice parameters of fcc Au ( a =4.078 Å, ICSD no. 52249) and fcc Ag ( a =4.086 Å, ICSD no. 604630) are almost the same (~0.2% mismatch), which is ideal for their epitaxial growth. Indeed, continuous lattice fringes from the Au core to the Ag shell were observed, indicating the epitaxial growth of the Ag shell on the Au core ( Fig. 2i and Supplementary Fig. 16 ). In addition, it was also observed that the insufficient coating of Ag can induce the formation of irregularly shaped and poorly crystallized Au@Ag nanostructures ( Supplementary Figs 18 and 19 ), which is consistent with that of ligand exchange ( Supplementary Fig. 6 ). 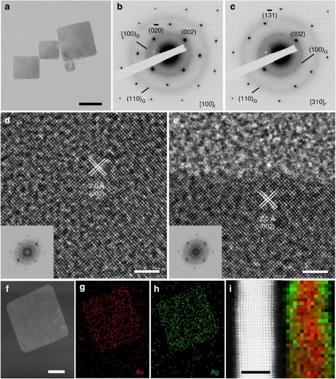Figure 2: TEM analysis of fcc Au@Ag square sheets. (a) Bright-field TEM image of fcc Au@Ag square sheets on GO surface prepared by coating Ag on hcp AuSSs with ascorbic acid as the reductant (scale bar, 100 nm). (b,c) SAED patterns of a typical fcc Au@Ag square sheet taken along the [100]fand [310]fzone axes, respectively. (d,e) HRTEM images of an fcc Au@Ag square sheet taken in the centre and on the edge areas, respectively (scale bars, 2 nm). (Insets) the corresponding FFT diffraction patterns of the HRTEM images shown indande. (f–h) HAADF–STEM image (scale bar, 50 nm) and the corresponding STEM–EDS elemental mappings of a typical fcc Au@Ag square sheet. (i) High-resolution HAADF–STEM image (scale bar, 2 nm) and the corresponding STEM–EDS elemental mapping of the cross-section of a typical fcc Au@Ag square sheet, revealing the Ag shell (green) and Au core (red). Figure 2: TEM analysis of fcc Au@Ag square sheets. ( a ) Bright-field TEM image of fcc Au@Ag square sheets on GO surface prepared by coating Ag on hcp AuSSs with ascorbic acid as the reductant (scale bar, 100 nm). ( b , c ) SAED patterns of a typical fcc Au@Ag square sheet taken along the [100] f and [310] f zone axes, respectively. ( d , e ) HRTEM images of an fcc Au@Ag square sheet taken in the centre and on the edge areas, respectively (scale bars, 2 nm). (Insets) the corresponding FFT diffraction patterns of the HRTEM images shown in d and e . ( f – h ) HAADF–STEM image (scale bar, 50 nm) and the corresponding STEM–EDS elemental mappings of a typical fcc Au@Ag square sheet. ( i ) High-resolution HAADF–STEM image (scale bar, 2 nm) and the corresponding STEM–EDS elemental mapping of the cross-section of a typical fcc Au@Ag square sheet, revealing the Ag shell (green) and Au core (red). Full size image Interestingly, when the reducing agent used for overgrowth of Ag on AuSS was changed to oleylamine instead of ascorbic acid or NaBH 4 , Au@Ag square sheets with the mixed hcp/fcc lattice structure were obtained ( Fig. 3 ). EDS analyses on both the plan-view and cross-sectional samples confirm the continuous coating of the Ag shell on Au core ( Supplementary Figs 20–23 ). XPS investigation indicates that the as-prepared Au@Ag square sheets are protected by oleylamine ( Supplementary Fig. 24 ). The thickness of the hcp/fcc Au@Ag square sheets was estimated to be 2.8±0.5 nm based on the cross-sectional TEM images ( Fig. 3e,g ; Supplementary Figs 23 and 25 ). A typical bright-field TEM image of the obtained Au@Ag square sheets is shown in Fig. 3a , which indicates that the edges of hcp AuSSs were slightly etched during the Ag-coating process. SAED pattern of such an Au@Ag square sheet ( Fig. 3b ) can be indexed as the hcp [110] h zone pattern together with diffuse diffraction spots streaking along the [001] h direction, indicative of the intergrowth of fcc and hcp phases together with stacking faults and twins along the [001] h /[111] f direction. This complex nanostructure was further revealed by the plan-view HRTEM images of the centre ( Fig. 3c ) and the edge ( Fig. 3d ) regions of an Au@Ag nanosheet (the hcp and fcc domains are highlighted), as well as the dark-field TEM image collected with the reflection ( Supplementary Fig. 26 ). To confirm the lattice relationship between the Ag shell and Au core, the Au@Ag nanosheets were cut along both the directions (see Supplementary Fig. 27 for the cutting direction) to reveal lattice patterns of the ( Fig. 3e ) and zones ( Fig. 3g ), respectively. From both the cross-sectional HAADF–STEM images and their corresponding fast Fourier transform (FFT) diffraction patterns ( Fig. 3e–h ), it can be clearly seen that the same atomic arrangement extends from the Au core to Ag shell, suggesting the coherent epitaxial growth. Note that from the viewing direction in Fig. 3g , and hcp(002) planes are superimposed, and therefore, the FFT pattern in Fig. 3h shows two sets of diffraction patterns, marked in red and green, respectively. 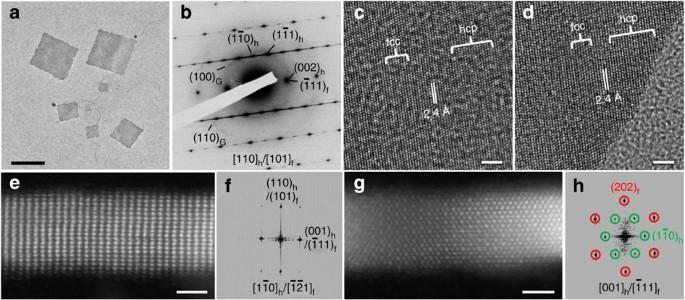Figure 3: TEM analysis of hcp/fcc Au@Ag square sheets. (a) Bright-field TEM image of hcp/fcc Au@Ag square sheets on GO surface (scale bar, 200 nm). (b) SAED pattern of a typical hcp/fcc Au@Ag square sheet along the [110]h/[101]fzone axis. (c,d) HRTEM images of a typical hcp/fcc Au@Ag square sheet taken in the centre and on the edge areas, respectively (scale bars, 2 nm). (e–h) High-resolution HAADF–STEM images (e,g) (scale bars, 1 nm) and the corresponding FFT diffraction patterns (f,h) of the cross-section of hcp/fcc Au@Ag square sheet taken along theand thezone axes, respectively. From the viewing direction in (g),and hcp(002) planes are superimposed, and therefore, its FFT pattern inhshows two sets of diffraction patterns, marked in red and green, respectively. Figure 3: TEM analysis of hcp/fcc Au@Ag square sheets. ( a ) Bright-field TEM image of hcp/fcc Au@Ag square sheets on GO surface (scale bar, 200 nm). ( b ) SAED pattern of a typical hcp/fcc Au@Ag square sheet along the [110] h /[101] f zone axis. ( c , d ) HRTEM images of a typical hcp/fcc Au@Ag square sheet taken in the centre and on the edge areas, respectively (scale bars, 2 nm). ( e – h ) High-resolution HAADF–STEM images ( e , g ) (scale bars, 1 nm) and the corresponding FFT diffraction patterns ( f , h ) of the cross-section of hcp/fcc Au@Ag square sheet taken along the and the zone axes, respectively. From the viewing direction in ( g ), and hcp(002) planes are superimposed, and therefore, its FFT pattern in h shows two sets of diffraction patterns, marked in red and green, respectively. 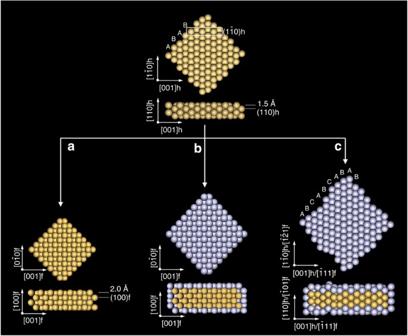Figure 4: Schematic illustration for the phase transformation of hcp AuSSs. The phase transformation of hcp AuSSs can be induced by (a) ligand exchange of oleylamine with ODT, (b) coating of Ag without oleylamine and (c) coating of Ag with oleylamine. Both the top view and cross-sectional side view are shown to illustrate the structures. Full size image Figure 4 schematically illustrates the phase transition of hcp AuSS induced by ligand exchange or coating of Ag. As shown in Fig. 4a , the ligand exchange of oleylamine with ODT induced the transformation of the initial (110) h -oriented hcp AuSS to the (100) f -oriented fcc Au nanosheet. This type of transformation can be realized via the relative sliding of adjacent (002) h planes in opposite directions, along with the simultaneous expansion of inter-plane spacing of (110) h planes and contraction of that of (002) h planes ( Supplementary Fig. 28 ) [40] , [41] , [42] . In addition, it can also be described as the flattening of planes (marked by the rectangle in the top image of Fig. 4 ), which is similar to the wurtzite-to-rock salt transformation pathway observed in some semiconductors, such as CdSe and GaN [40] , [41] , [42] . Figure 4: Schematic illustration for the phase transformation of hcp AuSSs. The phase transformation of hcp AuSSs can be induced by ( a ) ligand exchange of oleylamine with ODT, ( b ) coating of Ag without oleylamine and ( c ) coating of Ag with oleylamine. Both the top view and cross-sectional side view are shown to illustrate the structures. Full size image As for the phase transformation induced by the coating of Ag, when ascorbic acid or NaBH 4 was used as the reducing agent, the fcc Au@Ag nanosheet with (100) f orientation was obtained ( Fig. 4b ), similar to the fcc AuSS resulted from the ligand exchange ( Fig. 4a ). Note that the hcp AuSS initially capped with oleylamine was washed several times before being coated with Ag. Hence, only a small amount of oleylamine was left on the surface of AuSS. The second type of transformation, which occurred after coating Ag on hcp AuSS by using oleylamine as the only reducing and capping agent, perhaps belongs to the commonly observed Martensitic transformation ( Fig. 4c ). This type of transformation proceeds via the change of packing sequence of closed-packed planes, leading to the formation of stacking faults/twins or the mixed packing of hcp and fcc domains [21] . In addition, the orientation of nanostructure with respect to its close-packed direction (that is, [001] h and [111] f direction) is preserved before and after the phase transformation. The aforementioned observations imply that oleylamine played an important role in controlling the crystal structure of the final Au@Ag square sheets, that is, the formation of fcc (100) f -oriented or hcp/fcc (110) h /(101) f -oriented nanosheets. To further study the effect of surface ligands, we carried out control experiments by replacing oleylamine with octylamine (primary amine) or dioctylamine (secondary amine) as the reductant for deposition of Ag on hcp AuSSs while keeping all the other experimental conditions same. Our results showed that the octylamine-based reduction led to the formation of hcp/fcc Au@Ag nanosheets with (110) h /(101) f orientation ( Supplementary Fig. 29 ), similar to those obtained with oleylamine ( Fig. 3 ), whereas the reduction using dioctylamine resulted in the fcc (100) f -oriented structures ( Supplementary Fig. 30 ). Our observations suggested that primary amines may favour the formation of hcp-containing structures. This is consistent with previous reports demonstrating that primary amines favoured the formation of hexagonal wurtzite structures in certain semiconductors, such as GaP [43] . Therefore, the kind of capping agent used during coating of Ag facilitated the control over the type of phase transformation, which is likely caused by the interplay of the surfactant–metal bonding energy and the adhesive energy of the metal structures [44] , [45] . Monochromated EELS study of fcc AuSS and Au@Ag square sheet on GO The SPR property of a single fcc AuSS on GO was investigated by monochromated EELS (see Methods for details). Typically, the EELS measurement of a single fcc AuSS was conducted by locating the focused electron beam 2–3 nm next to the corner (or edge) of the AuSS on GO to excite its SPR ( Fig. 5a ). A reference EELS spectrum of GO was also collected ~500 nm away from the AuSS, where only GO is present ( Fig. 5b , blue curve). Interestingly, the EELS spectrum from the corner of AuSS on GO shows a strong peak at 0.59 eV (or 2,102 nm) ( Fig. 5b , red curve). The EELS spectrum from the edge of the AuSS on GO exhibits a similar SPR feature, which further confirms its SPR absorption in the infrared region ( Fig. 5b , green curve). Such strong infrared absorption can be attributed to the in-plane plasmon resonance of the two-dimensional AuSS with large aspect ratio (that is, edge length divided by thickness) [1] , [24] , [25] , [46] , [47] . Moreover, the SPR of a single fcc Au@Ag square sheet on GO was also measured by monochromated EELS, in which the measurement process is same as that for fcc AuSS. The reference EELS spectrum of GO was also collected ~500 nm away from the Au@Ag square sheet, where only GO is present ( Fig. 5c , blue curve). Remarkably, the EELS spectra of fcc Au@Ag square sheet on GO also display a strong peak at 0.61 eV (or 2,033 nm; Fig. 5c , red and green curves). 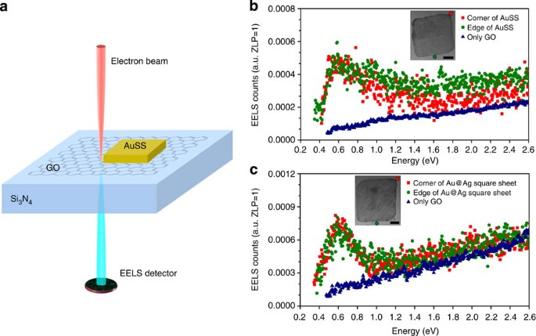Figure 5: SPR analysis of fcc AuSS and Au@Ag square sheet on GO. (a) Schematic illustration of monochromated EELS measurement of an individual fcc AuSS on GO. The focused electron beam is located next to the corner or edge of an AuSS to excite and measure its SPR. The monochromated EELS measurement process for fcc Au@Ag square sheet on GO is same as that for fcc AuSS. (b) EELS spectra acquired from AuSS on GO (excited next to the corner and edge of an AuSS) and GO. Inset: the corresponding bright-field STEM image of the measured AuSS on GO, in which the positions of the electron beam are marked (scale bar, 20 nm). (c) EELS spectra acquired from Au@Ag square sheet on GO (excited next to the corner and edge of an Au@Ag square sheet) and GO. Inset: the corresponding bright-field STEM image of the measured Au@Ag square sheet on GO, in which the positions of the electron beam are marked (scale bar, 20 nm). Figure 5: SPR analysis of fcc AuSS and Au@Ag square sheet on GO. ( a ) Schematic illustration of monochromated EELS measurement of an individual fcc AuSS on GO. The focused electron beam is located next to the corner or edge of an AuSS to excite and measure its SPR. The monochromated EELS measurement process for fcc Au@Ag square sheet on GO is same as that for fcc AuSS. ( b ) EELS spectra acquired from AuSS on GO (excited next to the corner and edge of an AuSS) and GO. Inset: the corresponding bright-field STEM image of the measured AuSS on GO, in which the positions of the electron beam are marked (scale bar, 20 nm). ( c ) EELS spectra acquired from Au@Ag square sheet on GO (excited next to the corner and edge of an Au@Ag square sheet) and GO. Inset: the corresponding bright-field STEM image of the measured Au@Ag square sheet on GO, in which the positions of the electron beam are marked (scale bar, 20 nm). Full size image In summary, we successfully achieve the phase transformation of AuSSs from hcp to fcc structures at ambient conditions via either ligand exchange or surface coating of a thin Ag layer. Significantly, the surfactants play an important role in controlling the type of phase transformation and thus the crystal structure and orientation of the final products. It is worth mentioning that noble metal nanosheets/nanoplates normally crystallize in the shape of hexagon or triangle, bound by low-energy {111} f basal planes [3] . The first study of fcc Au nanosheets with (111) f orientation dates back to the 1950s [48] . However, free-standing metal nanosheets with other orientations have not been achieved by wet-chemical method over the following decades. In the present work, the ~3-nm-thick (100) f -oriented fcc Au and Au@Ag nanosheets as well as the (110) h /(101) f -oriented hcp/fcc Au@Ag nanosheets are prepared. Remarkably, monochromated EELS identifies the strong infrared SPR absorption of the fcc AuSS and Au@Ag square sheet. It is believed that the method reported here will open up new opportunities towards the synthesis of novel metallic/bimetallic nanostructures, with potential applications in catalysis, electronics and plasmonics [1] , [3] . Chemicals Natural graphite (SP-1) was purchased from Bay Carbon (Bay City, MI). Gold(III) chloride hydrate (HAuCl 4 ·aq, ~52% Au basis), silver nitrate (AgNO 3 , ACS reagent, ≥99.0%), L -ascorbic acid (BioXtra, ≥99.0%, crystalline), KMnO 4 , H 2 SO 4 (98%), H 2 O 2 (30%), hexane (technical grade), oleylamine (70%, technical grade), octylamine (99%), ODT (98%) 1-dodecanethiol (DDT,≥98%), 1-octanethiol (OT, 98.5%), 1-propanethiol (PT, 99%), 11-mercapto-1-undecanol (MUDO, 98%), 6-mercapto-1-hexanol (MHO, 97%), 11-mercaptoundecanoic acid (MUDA, 95%), 3-mercaptopropionic acid (MPA, ≥99%), benzeneethanethiol (BET, 98%) and 1,6-hexanedithiol (HDT, ≥97%) were purchased from Sigma-Aldrich. Sodium borohydride (NaBH 4 , ≥99.0%) was purchased from Fluka. Concentrated hydrochloric acid (HCl, 37%) and ethanol (99.9%, absolute) were purchased from Merck. Ultrapure Milli-Q water (Milli-Q System, Millipore, Billerica, MA) was used in all the experiments. All the reagents were used as received without further purification. Synthesis of GO All the glassware was washed by aqua regia (HNO 3 /HCl=1:3, v/v) and then rinsed by Milli-Q water at least twice (caution: aqua regia is a quite strong oxidant and should be handled with great care). Single-layer GO sheets were synthesized from natural graphite by a modified Hummer’s method [49] . The as-prepared GO sheets were dispersed into ethanol with a concentration of 0.2 mg ml −1 by sonication. Synthesis of hcp AuSSs on GO The AuSSs were synthesized following our recently reported method with a slight modification [28] . Typically, GO in ethanol (0.2 mg ml −1 , 200 μl) was centrifuged and re-dispersed into a 2 ml growth solution containing 7.25 mM HAuCl 4 and 150 mM oleylamine in a mixed solvent of hexane and ethanol (7/1, v/v). Then, the 2 ml growth solution in a capped glass vial was heated in a water bath at 58 °C for 16 h. After that, the final product was purified by centrifugation (5,000 r.p.m., 5 min) for four times and then re-dispersed in 2.0 ml of hexane. Ligand exchange on hcp AuSSs Equal volumes of the as-prepared hcp AuSS solution (concentration of Au atoms of ~4.6 mM in hexane) and a fresh thiol (for example, ODT, DDT, OT, PT, MUDO, MHO, MUDA, MPA, BET and HDT, see Supplementary Fig. 9 for details) solution (50 mM in hexane) were mixed together and then vortexed for 5 min. After that, the solution was centrifuged for two times and the sediments were re-dispersed in hexane before further characterizations. To investigate the effect of thiol concentration, ODT solutions with different concentrations ranging from 2 to 200 mM were used for the ligand exchange while the other experimental conditions were kept same. Preparation of fcc Au@Ag square sheets The fcc Au@Ag square sheets were prepared through the epitaxial seeded growth of Ag on hcp AuSSs by using L -ascorbic acid (or NaBH 4 ) as the reducing agent. Typically, 350 μl of ethanol and 50 μl of AgNO 3 solution (4 mM, ethanol) were firstly added into 500 μl of the as-prepared hcp AuSSs solution (hexane) in turn. The mixture was gently shaken and cooled in a water-ice bath. After that, 100 μl of 1 mM L -ascorbic acid in ethanol (or 0.5 mM NaBH 4 in ethanol) was quickly added into the above mixture, followed by gentle shaking. The final growth solution was then kept undisturbed in the water-ice bath for 2 h. The product was collected by centrifugation (8,000 r.p.m., 1 min) and washed once with hexane before further characterization. Preparation of hcp/fcc Au@Ag square sheets The hcp/fcc Au@Ag square sheets were synthesized through the epitaxial seeded growth of Ag on hcp AuSSs by using oleylamine as the reducing agent. Typically, 133 μl of oleylamine, 230 μl of ethanol, 20 μl of AgNO 3 solution (20 mM, ethanol) and 620 μl of hexane were added into 1.0 ml of the as-prepared hcp AuSSs solution (hexane) in turn. Then the glass vial containing the above growth solution was sealed and heated in a water bath at 38 °C for 20 h. The product was collected by centrifugation (5,000 r.p.m., 2 min) and washed twice with hexane before further characterization. Fabrication of the cross-section samples of fcc AuSSs and Au@Ag square sheets Cross-sectional samples of fcc AuSSs and Au@Ag square sheets were prepared on an FEI Nova NanoLab 600i focused ion beam (FIB)/SEM dual-beam system, using tungsten (W) deposition for sample protection. Typically, fcc AuSSs and Au@Ag square sheets were first pre-deposited on a silicon substrate and dried in air. After the sample was inserted into the SEM chamber, a typical fcc AuSS or Au@Ag square sheet of interest was located and rotated so that one of its two diagonals (equal to each other) was parallel to the horizontal x axis of the SEM system. A thin layer of W was then deposited on the area of interest with electron beam-induced deposition. Next, two alignment marks were milled to identify the position of the interested area before further deposition of a W protective layer with FIB. After that, the region of interest was transferred to a TEM half-grid using an in situ manipulator, followed by final thinning of the sample with FIB. Fabrication of the cross-section samples of hcp/fcc Au@Ag square sheets Cross-sectional samples of hcp/fcc Au@Ag square sheets were prepared on an FEI Helios NanoLab 400S FIB/SEM dual-beam system, using Pt/C deposition for sample protection. Note that the two diagonals of hcp/fcc Au@Ag square sheets are not equal to each other, cross-section samples are prepared by cutting along both and directions, respectively (See Supplementary Fig. 27 for details). Typically, hcp/fcc Au@Ag square sheets were first pre-deposited on a silicon substrate and dried in air. After the sample was inserted into the SEM chamber, a typical hcp/fcc Au@Ag square sheet of interest was located and rotated so that one of its diagonals (unequal to each other) was parallel to the horizontal x axis of the SEM system. A thin layer of C was then deposited on the area of interest with electron beam-induced deposition. Next, two alignment marks were milled to identify the position of the area of interest before further deposition of a Pt protective layer with FIB. After that, the region of interest was transferred to a TEM half-grid using an in situ manipulator, followed by final thinning of the sample with FIB. SPR characterization of both fcc AuSS and Au@Ag core-shell square sheet Monochromated EELS study of single sheets was conducted in STEM mode using an FEI Titan TEM with Schottky electron source, operated at a selected voltage of 80 kV, using a convergence semiangle of 13 mrad and a collection semiangle of 20 mrad. The diameter of the used electron probe was around 1 nm and an energy resolution of 70 meV was obtained by using a Wien-type monochromator. In this way, an EELS spectrum was acquired from an individual sheet on GO, by locating the focused incident electron beam 2–3 nm next to the single sheet for exciting and detecting its SPR. A reference spectrum was also obtained ~500 nm away from the single sheet, with only the GO component present and without exciting the SPR of the single sheet. The acquisition time was set as 1 s to avoid the effect of organic contamination. Because of the rather short acquisition time, the final signal-to-noise ratio of the EELS spectra is relatively low. Characterization The TEM samples were prepared by directly dropping ~5 μl of sample solution onto full carbon-coated copper grid (200 mesh) and dried under ambient conditions. TEM images were collected by a JEOL JEM-2010 TEM operated at 200 kV. HRTEM images, SAED patterns and the HAADF–STEM–EDS data were taken on a JEOL JEM-2100F TEM operated at 200 kV. To characterize the cross-sectional samples, high-resolution STEM was performed on an FEI aberration-corrected Titan Cubed S-Twin TEM operated at 300 kV. Probe Cs corrector was applied to get better spatial resolution. In a typical experiment, high-resolution STEM imaging was conducted at a 20 μs per pixel scanning rate with 50 μm C2 aperture, spot size 7, a HAADF detector, and 146-mm camera length. Under such conditions, a spatial resolution of ~1.0 Å was obtained. The oxidation state of Au and S in the obtained fcc AuSSs is measured by XPS(AXIS ultra spectrometer, Kratos). How to cite this article: Fan, Z. et al . Surface modification-induced phase transformation of hexagonal close-packed gold square sheets. Nat. Commun , 6:6571 doi: 10.1038/ncomms7571 (2015).